Evolutionary expansion of a regulatory network by counter-silencing Horizontal gene transfer plays a major role in bacterial evolution. Successful acquisition of new genes requires their incorporation into existing regulatory networks. This study compares the regulation of conserved genes in the PhoPQ regulon of Salmonella enterica serovar Typhimurium with that of PhoPQ-regulated horizontally acquired genes, which are silenced by the histone-like protein H-NS. We demonstrate that PhoP upregulates conserved and horizontally acquired genes by distinct mechanisms. Conserved genes are regulated by classical PhoP-mediated activation and are invariant in promoter architecture, whereas horizontally acquired genes exhibit variable promoter architecture and are regulated by PhoP-mediated counter-silencing. Biochemical analyses show that a horizontally acquired promoter adopts different structures in the silenced and counter-silenced states, implicating the remodelling of the H-NS nucleoprotein filament and the subsequent restoration of open-complex formation as the central mechanism of counter-silencing. Our results indicate that counter-silencing is favoured in the regulatory integration of newly acquired genes because it is able to accommodate multiple promoter architectures. Horizontal gene transfer is a primary driver of evolution in bacteria [1] . However, the simple acquisition of a gene encoding a beneficial trait, such as virulence or antibiotic resistance, is insufficient to improve the fitness of the bacterial cell. For the potential benefit of a newly acquired gene to be realized by the host cell, the gene must be expressed in a physiologically and environmentally appropriate manner. Unchecked expression of a newly acquired gene may be energetically and physiologically costly, placing a recipient cell at a competitive disadvantage. This can be avoided via a phenomenon termed xenogeneic silencing [2] , wherein horizontally acquired DNA is recognized and transcriptionally silenced by a class of DNA-binding proteins, represented by the archetypal histone-like nucleoid-structuring protein (H-NS) in Salmonella Typhimurium [2] , [3] , [4] . H-NS, as well as analogous proteins in other species such as Lsr2 in Mycobacterium tuberculosis [5] and MvaT in Pseudomonas aeruginosa [6] , preferentially silences foreign DNA with increased AT content relative to the resident genome [2] , [3] , [7] . This activity is attributed to H-NS binding via a conserved Q/RGR motif to the minor groove of DNA [8] . H-NS–protein interactions favour AT-rich sequences [9] , [10] and permit subsequent polymerization and spreading of H-NS along adjacent regions of DNA to inhibit gene expression [11] . H-NS polymerization and silencing is dependent on the nature of the H-NS–DNA interaction, which occurs in two possible modes: a ‘bridging’ mode, in which H-NS binds and links distant DNA sequences in parallel to form DNA loops [12] , and a ‘stiffening’ mode, in which H-NS increases DNA rigidity upon binding to form a stiff nucleoprotein filament [13] . In the cell, H-NS binding is thought to alternate between these two modes in an environmentally and physiologically responsive manner [14] , modulating H-NS activity as required. The silencing of foreign DNA by an H-NS-type silencer is only one step in the process of integrating a newly acquired gene into the host genome. Ultimately, for a new gene to be faithfully maintained by a recipient cell, it must also evolve a regulatory circuit to allow timely and appropriate expression that confers a competitive advantage. It is unknown whether this occurs by the evolution of a classical transcription activation circuit, which is typically envisaged as a process in which a DNA-binding protein binds specific sequences near a promoter and recruits RNA polymerase (RNAP) to result in increased transcription [15] , as in CAP-mediated activation of the lac operon [16] , or a counter-silencing circuit, wherein DNA-binding proteins oppose the activity of H-NS-type silencers to relieve repression and allow transcription. In fact, it is unclear whether these are separate mechanisms at all, as activation and counter-silencing have not been distinguished at a mechanistic level. However, the classical activation model presents an additional obstacle to successful integration of horizontally acquired genes; an activator must bind in the appropriate position and orientation relative to a target promoter so as to allow direct appropriate interaction with RNAP. Despite this, many bacterial transcription factors appear to act at promoters possessing a variety of architectures, binding in either orientation and at a wide array of positions relative to the promoter. This observation raises the questions of how a simple transcriptional activator is able to act within the context of such varied architectures and whether promoter arrangements correspond to distinct regulatory mechanisms. In this study, we use the model PhoPQ two-component signal transduction system in S. Typhimurium to examine the distinction between activation and counter-silencing. The OmpR-family transcriptional activator PhoP is essential for Salmonella virulence [17] , [18] and exemplifies a regulatory protein capable of acting at a variety of promoter architectures [19] . Phosphorylation by the sensor kinase PhoQ in response to low extracellular Mg 2+ concentrations or antimicrobial peptides at acidic pH [20] , [21] allows PhoP to bind to specific promoters, resulting in transcriptional upregulation ( Fig. 1a ). PhoP is able to upregulate both horizontally acquired and core genes possessing a wide variety of promoter architectures, but the mechanistic details of PhoP actions at different types of promoter are poorly understood. Previous studies have failed to identify any distinction between counter-silencing and activation by PhoP, and some investigators have suggested that PhoP is able to activate transcription at multiple target architectures [19] , [22] , [23] . 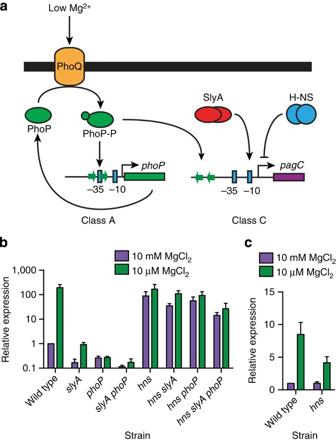Figure 1: Genetic analysis of PhoP-regulated circuits. (a) PhoP is activated via phosphorylation by the membrane-associated sensor kinase, PhoQ, in response to low extracellular Mg2+or cationic antimicrobial peptides at acidic pH. Phosphorylated PhoP (PhoP-P) upregulatesphoPandpagC. Upregulation ofpagCalso requires SlyA and repression by H-NS. RT–PCR analysis ofpagC(b) andphoP(c) mRNA under inducing (10 μM Mg2+) and non-inducing (10 mM Mg2+) conditions. Data represent the mean±s.e.m.;n=3. Other PhoP regulon members gave similar results (Supplementary Fig. 1). Figure 1: Genetic analysis of PhoP-regulated circuits. ( a ) PhoP is activated via phosphorylation by the membrane-associated sensor kinase, PhoQ, in response to low extracellular Mg 2+ or cationic antimicrobial peptides at acidic pH. Phosphorylated PhoP (PhoP-P) upregulates phoP and pagC . Upregulation of pagC also requires SlyA and repression by H-NS. RT–PCR analysis of pagC ( b ) and phoP ( c ) mRNA under inducing (10 μM Mg 2+ ) and non-inducing (10 mM Mg 2+ ) conditions. Data represent the mean±s.e.m. ; n =3. Other PhoP regulon members gave similar results ( Supplementary Fig. 1 ). Full size image Here we demonstrate that activation and counter-silencing are separate mechanisms of transcription regulation with distinctive promoter architecture. Classically activated promoters are structurally constrained, with a PhoP-binding site precisely overlapping the −35 box of the promoter, whereas counter-silenced promoters exhibit an array of architectures at which PhoP acts by disrupting silencing. Activated promoters are highly conserved members of the PhoP core regulon, whereas counter-silenced promoters are typically horizontally acquired Salmonella -specific genes, suggesting an evolutionary pathway by which horizontally acquired genes can achieve regulatory integration in a new host. Biochemical analysis of the counter-silenced pagC promoter shows that PhoP and SlyA cooperatively induce DNA bending in an H-NS-bound region upstream of the pagC promoter to restore open-complex formation by RNAP. Architectural classification of PhoP targets A set of 23 PhoP targets were previously defined on the basis of promoter architecture [19] . The previous study indicated that PhoP acts on an array of different architectures and suggested that some might represent different mechanisms of transcription regulation. In view of its ability to oppose the regulatory actions of H-NS as well as function as a classical activator [23] , we hypothesized that promoter architecture might be a primary determinant of whether PhoP acts as an activator or counter-silencer. To address this possibility, we analysed these targets with respect to their binding by H-NS [2] ( Table 1 ). Group A promoters have a single PhoP-binding site overlapping the −35 box, whereas group B promoters have a single PhoP-binding site immediately upstream of the −35 box. Group C promoters are defined by a PhoP-binding site with variable distance and orientation upstream of the −35 box, as well as additional distant binding sites, although in the case where there is only one PhoP-binding site at a group C promoter, it appears to be in the reverse orientation ( Supplementary Fig. 1 ). Other promoters represent hybrids of groups A and C or groups B and C. Table 1 PhoP regulon promoter architecture. Full size table Of these 23 genes, all but six are bound by H-NS, and five of these H-NS-independent loci belong to group A. The average AT content of the coding sequences of group A genes is 48%, which is identical to that of the S . Typhimurium genome overall, in contrast to the 53% mean AT content of the 23 PhoP-activated genes. This suggests that the PhoP regulon in S . Typhimurium is largely horizontally acquired and Salmonella -specific, whereas group A genes are shared among multiple species, representing the core PhoP regulon. This conclusion is supported by the conservation of all but one group A gene ( orgB ) in both S. Typhimurium 14028s and Escherichia coli K-12, a close relative of S . Typhimurium with respect to the PhoP regulon [19] . In contrast, only four out of 15 Salmonella genes with group C or hybrid promoter architectures are found in E. coli . Based on these observations, we hypothesized that classical activation via PhoP occurs at group A genes, independent of H-NS and requiring a binding site overlapping the −35 box. Conversely, we hypothesized that H-NS-dependent counter-silencing might be occurring at the non-group A genes, and that PhoP antagonism of H-NS-mediated silencing is considerably less structurally constrained, allowing for greater variability in promoter architecture. H-NS and PhoP-mediated regulation of PhoP regulon members To test these hypotheses, genetic analyses were performed on the 14 single-group (A, B or C) PhoP regulon members described in Table 1 . Transcript levels were quantified for each gene under non-inducing (high Mg 2+ minimal medium) and inducing (low Mg 2+ minimal medium) conditions in wild-type, phoP , hns and hns phoP strains. Of these 14 genes, 11 were significantly induced (>5-fold) in low Mg 2+ medium ( Supplementary Fig. 2 ). Data from two representative PhoP targets, the phoP and pagC promoters, are shown in Fig. 1 . The model phoP promoter is a member of the core PhoP regulon [19] exhibiting group A architecture. Transcription of phoP is upregulated in low Mg 2+ minimal medium in both wild-type and hns strains, indicating that PhoP acts as an H-NS-independent regulator of phoP ( Fig. 1c ). Only one of the other group A genes, orgB , failed to fit this model. orgB expression is derepressed in an hns mutant and is not upregulated in low Mg 2+ medium. However, this does not exclude the possibility of classical PhoP-mediated activation of orgB , as transcription may become saturating in the absence of H-NS. The other two group A genes, mgtA and pmrD , were both expressed in a manner fitting this model, although mgtA also exhibited PhoP-independent, Mg 2+ -dependent regulation, likely via a Mg 2+ -sensitive region of the 5′ untranslated region of mgtA [24] . The prototypical group C promoter, pagC , regulates a horizontally acquired virulence gene used as a model for H-NS silencing in S . Typhimurium [23] . PhoP, along with SlyA, a virulence-associated DNA-binding protein, cooperatively opposes H-NS silencing at the pagC promoter ( Fig. 1a ). pagC is upregulated upon growth in low Mg 2+ minimal medium but is also derepressed in an hns mutant strain ( Fig. 1b ). Disruption of either phoP or slyA results in an inability to overcome H-NS-mediated repression and an overall decrease in pagC expression. However, neither a slyA nor a phoP mutation has a significant effect on pagC induction in an hns mutant background, suggesting that the sole in vivo function of both PhoP and SlyA at the pagC promoter is to counter H-NS. None of the group B or C promoters described in Table 1 were significantly activated by PhoP in an hns mutant background, further supporting this hypothesis ( Supplementary Fig. 2 ). However, one group C gene, mgtC , exhibited H-NS- and PhoP-independent, Mg 2+ -dependent control [25] , and the hns mutation appeared to be epistatic to phoP for group B genes. Although an hns mutation does not de-repress group B genes, PhoP is no longer able to activate these promoters, suggesting indirect regulation via additional factors. PhoP-mediated activation requires class A architecture As we were unable to a make a direct correlation between promoter architecture and the mechanism of PhoP-mediated control based on the genetic data alone, owing to the complex nature of these circuits in vivo , PhoP activity was directly interrogated at each promoter using in vitro transcription (IVT) assays on all 11 PhoP targets described in Fig. 1 and Supplementary Fig. 2 ( Fig. 2 ). Previous studies have observed PhoP-mediated activation at a variety of promoter architectures, including pagC , ugtL and rstA , an observation which is not corroborated by our in vivo reverse transcription PCR (RT–PCR) data ( Fig. 1 and Supplementary Fig. 2 ). However, earlier studies have used short linear fragments as templates [19] , [23] , which may not resemble the physiological PhoP target in the bacterial cell. As supercoiling has been shown to have a significant impact on regulation by both OmpR-family two-component system response regulators [26] and H-NS [27] , we hypothesized that short linear fragments, which do not resemble the larger, supercoiled chromosome, might be yielding non-physiological results. We therefore carried out IVT assays using supercoiled templates carrying large (≥2 kb) fragments of the target promoter regions to maintain appropriate structure and context, and quantified transcripts by quantitative RT–PCR(qRT–PCR) using sequence- and strand-specific probes (see Methods section). This ensured unambiguous identification and quantification of mRNA, as compared with more traditional radioisotope-labelled transcription run-off experiments, which are unable to assign and confirm the specific sequence identities of transcription products. In contrast to earlier findings using smaller linear DNA [23] , our IVT analyses revealed that only group A promoters are significantly activated by phosphorylated PhoP (PhoP-P). Three of the four group A genes examined ( mgtA , orgB and phoP ) were activated >2-fold by PhoP-P. Notably, orgB is activated despite having a high AT content (55%). This indicates that architecture, rather than AT content, determines whether PhoP is able to activate a promoter. The position of the PhoP-P-binding site was confirmed via DNase I footprinting for the model group A gene, phoP ( Supplementary Fig. 3 ), and the target promoter was confirmed via site-directed mutagenesis of the phoP promoter in IVT assays ( Supplementary Fig. 4a ). Transcription of the fourth group A gene, pmrD , was still activated, but not as strongly as other group A promoters, likely owing to pmrD possessing only one half of the tandem repeat consensus PhoP-binding sequence [28] . As pmrD exhibits a higher AT content (52%) than the average group A gene (48%), we posit that pmrD may have been more recently acquired than other group A genes and thus has not yet evolved a strong consensus PhoP-binding site. None of the group B or C genes tested exhibited significant (>2-fold) PhoP-P-dependent activation. 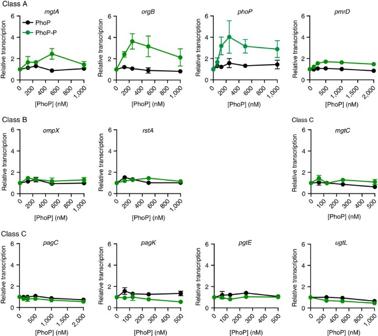Figure 2: PhoP-mediated activation is dependent on promoter architecture. IVT was performed on each of the PhoP target genes described inFig. 1andSupplementary Fig. 1in the presence of increasing concentrations of PhoP (black line) and PhoP-P (green line). Only class A genes are activated by PhoP-P. Transcriptional output is normalized to the 0-nM reaction. Data represent the mean±s.e.m.;n=3 for all genes exceptompX,pagKandrstA, wheren=4. Figure 2: PhoP-mediated activation is dependent on promoter architecture. IVT was performed on each of the PhoP target genes described in Fig. 1 and Supplementary Fig. 1 in the presence of increasing concentrations of PhoP (black line) and PhoP-P (green line). Only class A genes are activated by PhoP-P. Transcriptional output is normalized to the 0-nM reaction. Data represent the mean±s.e.m. ; n =3 for all genes except ompX , pagK and rstA , where n =4. Full size image In order to address the discrepancy between our IVT results using large supercoiled templates and previous studies that used linear templates, we performed IVT analysis of the pagC promoter region using a 300-base pair (bp) DNA fragment identical to that described by Perez et al . [23] , with the transcription start site (TSS) located 122 bp from the terminus ( Supplementary Fig. 5 ). As an additional control, we included a 300-bp fragment of the phoP promoter region with the TSS 122 bp from the terminus. We observed at least seven major pagC -related transcript species, five of which were activated by PhoP-P. The remaining two major species appear to be repressed by PhoP-P. These observations suggest that multiple cryptic promoters are active on the linear pagC promoter fragment, and that PhoP-P regulates them non-specifically. We confirmed the activation of pagC transcription on linear templates using RT–PCR-based quantification ( Supplementary Fig. 5c ). This indicated that the discrepancy was likely owing to the use of a small linear template rather than a difference in the quantification method. Interestingly, the linear phoP promoter region exhibited only low levels of activation when compared with linear pagC and supercoiled phoP . This casts further doubt on the accuracy of IVT assays using small fragments, as phoP represents the prototypical PhoP target and should exhibit robust activation. Given that neither the results for linear pagC nor linear phoP are corroborated by in vivo qRT–PCR measurements ( Fig. 1 ), we suggest that, at least in the case of PhoP, small linear fragments are less physiologically representative than supercoiled templates of the conditions in intact cells. To test the hypothesis that PhoP-P acts as a counter-silencer rather than as an activator at non-group A genes, we reconstituted a counter-silencing circuit in vitro using the model group C pagC gene. To confirm the role of H-NS as a specific repressor of pagC , IVT analyses were performed on pagC in the presence of increasing H-NS concentrations. The transcriptional output of pagC decreased by more than 10-fold in the presence of 600 nM H-NS, whereas the group A phoP gene was only modestly repressed ( Fig. 3a ). Neither PhoP-P nor SlyA alone was capable of relieving H-NS silencing, whereas the two proteins in combination increased pagC transcription ( Fig. 3b and Supplementary Fig. 4b ). This increase was not because of the formation of a SlyA-PhoP-P activator complex, as no increase in mRNA was detectable in the absence of H-NS ( Fig. 3c ), indicating that PhoP acts as a counter-silencer of pagC via a mechanism distinct from the classical transcriptional activation observed at the phoP promoter. 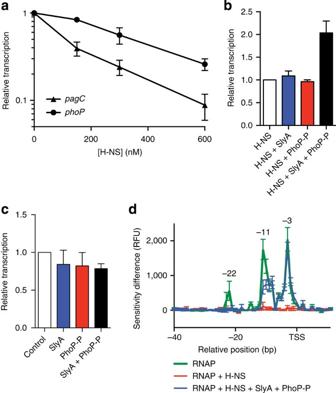Figure 3: Reconstitution of thepagCcounter-silencing circuitin vitro. (a) H-NS strongly repressespagC in vitro. Transcriptional outputs are normalized to the 0 nM control reaction. (b) Reconstitution ofpagCcounter-silencingin vitro. ApagC-containing template was incubated in the presence of 600 nM H-NS, 100 nM SlyA and 500 nM PhoP-P, as indicated. Transcriptional output is normalized to the H-NS reaction. Both SlyA and PhoP-P are required for counter-silencing. (c) SlyA and PhoP-P do not act as co-activators in the absence H-NS. ApagC-containing template was incubated in the presence of 100 nM SlyA, 500 nM PhoP-P (Fig. 2) or both as indicated. Transcriptional output is normalized the control reaction. Data represent the mean±s.e.m.;n=3. (d) KMnO4footprinting analysis indicates that RNAP is unable to form an open complex in the presence of H-NS. The addition of SlyA and PhoP-P restores open-complex formation at thepagCpromoter. Results are presented as a DDFA plot representing difference in peak height in relative fluorescent units (RFUs) between the control (no RNAP) and the experimental samples. Peaks indicate regions of single-stranded DNA caused by open-complex formation. The relative distance to the transcriptional start site (TSS) is indicated on the horizontal axis. Data represent the mean±s.d.;n=3. See alsoSupplementary Figs 3and4. Figure 3: Reconstitution of the pagC counter-silencing circuit in vitro . ( a ) H-NS strongly represses pagC in vitro . Transcriptional outputs are normalized to the 0 nM control reaction. ( b ) Reconstitution of pagC counter-silencing in vitro . A pagC -containing template was incubated in the presence of 600 nM H-NS, 100 nM SlyA and 500 nM PhoP-P, as indicated. Transcriptional output is normalized to the H-NS reaction. Both SlyA and PhoP-P are required for counter-silencing. ( c ) SlyA and PhoP-P do not act as co-activators in the absence H-NS. A pagC -containing template was incubated in the presence of 100 nM SlyA, 500 nM PhoP-P ( Fig. 2 ) or both as indicated. Transcriptional output is normalized the control reaction. Data represent the mean±s.e.m. ; n =3. ( d ) KMnO 4 footprinting analysis indicates that RNAP is unable to form an open complex in the presence of H-NS. The addition of SlyA and PhoP-P restores open-complex formation at the pagC promoter. Results are presented as a DDFA plot representing difference in peak height in relative fluorescent units (RFUs) between the control (no RNAP) and the experimental samples. Peaks indicate regions of single-stranded DNA caused by open-complex formation. The relative distance to the transcriptional start site (TSS) is indicated on the horizontal axis. Data represent the mean±s.d. ; n =3. See also Supplementary Figs 3 and 4 . Full size image Biochemical analyses of PhoP-mediated counter-silencing Little mechanistic data are available on how counter-silencing might occur, but previous studies have suggested that counter-silencing by PhoP and SlyA does not dissociate H-NS from the pagC promoter [23] . Therefore, counter-silencing might involve a structural change at the DNA level that allows RNAP binding despite the presence of H-NS. To observe the structural changes associated with counter-silencing, we performed differential DNA footprint analysis (DDFA) of DNase I, KMnO 4 , and ultraviolet laser footprinting under universal reaction conditions. Reactions for each experiment were assembled under the same conditions as used for the IVT experiments, allowing the correlation of discrete structural states of the pagC promoter region to specific transcriptional outputs. KMnO 4 analysis, which detects regions of single-stranded DNA associated with RNAP binding and open-complex formation [29] , suggested that the pagC promoter alone is transcriptionally competent, as stable open complexes were detected when RNAP was added in the absence of other factors ( Fig. 3d and Supplementary Fig. 6 ). However, detectable open-complex formation was completely inhibited by the addition of H-NS. This suggests that H-NS does not repress the pagC promoter by trapping RNAP [30] as a result of binding to sites both upstream and downstream of the promoter to form a repressive loop that surrounds the open complex, but rather inhibits pagC transcription by occluding the promoter to prevent RNAP binding, as shown for the E. coli proU and bgl promoters [31] , [32] . Addition of the counter-silencing proteins SlyA and PhoP-P restored open-complex formation at the pagC promoter, suggesting that RNAP binding and open-complex formation is a potential rate-limiting step at a silenced pagC promoter. However, when H-NS is absent, PhoP-P increases open-complex formation at both pagC and phoP , suggesting that PhoP-P can also recruit RNAP to naked promoters ( Supplementary Fig. 7 ). This does not by itself result in an increase in pagC transcription, suggesting that open-complex formation is not rate-limiting for transcription in the absence of H-NS. This is further supported by genome-wide studies in E . coli , which demonstrate that many silent promoters are bound by RNAP, and that the rate-limiting step in the transcriptional process is often downstream of RNAP binding [33] . Thus, although PhoP-P is capable of promoting open-complex formation at pagC , neither PhoP-P nor SlyA are necessary for transcription unless H-NS is present; rather, these proteins facilitate RNAP binding in the presence of H-NS. DNase I footprinting shows that H-NS binds extensively to the promoter region under silencing conditions (−117 to +16) ( Fig. 4 and Supplementary Fig. 8 ). PhoP binds to a discrete site located between positions −83 and −60, resulting in two hypersensitive sites at −70 and −68. Increases in sensitivity to DNase I-mediated cleavage are typically the result of a distortion or bend in the DNA duplex, resulting in the extrusion and increased digestion of individual bases, suggesting that PhoP induces the formation of a bend at this site. SlyA binds extensively across the pagC promoter region, (protected sites at −117, −104, −83, −35 and −11), as well as downstream of the H-NS-bound region at +59. SlyA also induces a modest change in sensitivity near position −83, which overlaps the promoter-distal half of the PhoP-binding site. Increases in sensitivity are observed at −38 and +35, indicating that SlyA binding also bends or distorts the DNA duplex. 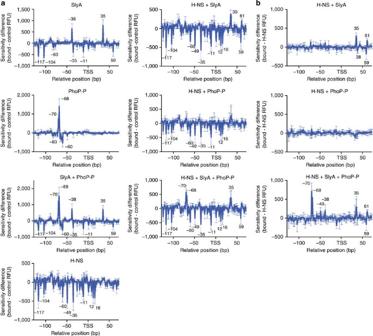Figure 4: DNase I DDFA of thepagCpromoter region. In vitroDNase I footprinting studies were performed on thepagCpromoter region with H-NS, SlyA and PhoP-P at concentrations of 600, 100 and 500 nM, respectively, as indicated. DNA–protein complexes were incubated at room temperature before digestion with DNase I. Results are presented as DDFA plots, representing the difference in fluorescent peak height (relative fluorescent unit, RFU) between the protein-free control and the experimental sample (a). DDFA plots are also shown for the H-NS+SlyA, H-NS+PhoP-P and H-NS+SlyA+PhoP-P reactions, representing the difference between the H-NS control and the experimental sample (b). The relative distance in base pairs to the TSS is indicated on the horizontal axis. Peaks indicate regions of hypersensitivity, typical of bent or distorted DNA, whereas valleys indicate protected regions, typical of protein binding sites. Approximate sizes of peaks of note are indicated. Data represent the mean±s.d.;n=3. SeeSupplementary Fig. 5for representative raw chromatograms. Figure 4: DNase I DDFA of the pagC promoter region. In vitro DNase I footprinting studies were performed on the pagC promoter region with H-NS, SlyA and PhoP-P at concentrations of 600, 100 and 500 nM, respectively, as indicated. DNA–protein complexes were incubated at room temperature before digestion with DNase I. Results are presented as DDFA plots, representing the difference in fluorescent peak height (relative fluorescent unit, RFU) between the protein-free control and the experimental sample ( a ). DDFA plots are also shown for the H-NS+SlyA, H-NS+PhoP-P and H-NS+SlyA+PhoP-P reactions, representing the difference between the H-NS control and the experimental sample ( b ). The relative distance in base pairs to the TSS is indicated on the horizontal axis. Peaks indicate regions of hypersensitivity, typical of bent or distorted DNA, whereas valleys indicate protected regions, typical of protein binding sites. Approximate sizes of peaks of note are indicated. Data represent the mean±s.d. ; n =3. See Supplementary Fig. 5 for representative raw chromatograms. Full size image In the presence of H-NS, neither SlyA nor PhoP-P was observed to bind upstream of the promoter in the H-NS-bound region, although SlyA binding was observed downstream of the promoter at +59. However, under counter-silencing conditions, SlyA and PhoP-P act cooperatively to form the PhoP-P-induced bend at −70 and −68, with additional sensitive sites at −49 and −38. Strikingly, most H-NS was not displaced despite pronounced changes in the structure of the nucleoprotein complex. Ultraviolet laser footprinting, wherein a high-intensity ultraviolet (266 nm) laser pulse probes DNA structural changes in response to protein binding [34] , suggests that H-NS-dependent structural changes are limited to a discrete region upstream of the TSS (−111 to −43), henceforth referred to as the upstream regulatory region (URR) ( Fig. 5 and Supplementary Fig. 9 ). Decreased crosslinking in the URR suggests fewer intramolecular contacts between adjacent bases, consistent with the ‘stiffening’ mode of H-NS binding [14] . As recent studies indicate that stiffening is required for silencing [35] , the structure of the URR may be important for the regulation of pagC transcription. Although both proteins altered the URR structure in the absence of H-NS, neither PhoP nor SlyA alone were capable of altering the URR structure in the presence of H-NS. However, SlyA was observed by DNase I footprinting to bind DNA downstream of the TSS (+38 to +59) and outside of the H-NS-bound region independently of PhoP-P. Under counter-silencing conditions, PhoP appeared to act cooperatively with SlyA to alter the URR structure at −84 and −77, resembling SlyA-bound DNA at those sites in the absence of H-NS. These results corroborate and extend the findings of the DNase I footprinting analysis, demonstrating that counter-silencing of pagC results when SlyA alters the structure of H-NS-bound DNA in the URR, thereby allowing PhoP-P to bend the DNA and to facilitate open-complex formation. 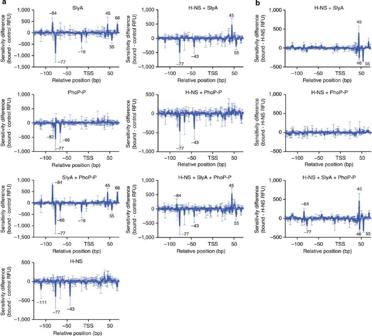Figure 5: Ultraviolet laser DDFA of thepagCpromoter region. Plasmid DNA containing thepagCregion was incubated in the presence of 600 nM H-NS, 100 nM SlyA and 500 nM PhoP-P as indicated and exposed to a single pulse of 266 nm radiation. Crosslinking was quantified by fluorescent primer extension. The relative distance to the TSS is indicated in base pairs on the horizontal axis. Results are presented as DDFA plots, representing the difference in fluorescent peak height (relative fluorescent unit, RFU) between the protein-free control and the experimental sample (a). DDFA plots are also shown for the H-NS+SlyA, H-NS+PhoP-P and H-NS+SlyA+PhoP-P reactions representing the difference between the H-NS control and the experimental sample (b). Peaks represent a protein-induced change in DNA structure, typically owing to increased intramolecular contacts or DNA–protein crosslinks. Valleys also represent a change in DNA structure owing to decreased intramolecular contacts. Approximate sizes of peaks of note are indicated. Data represent the mean±s.d.;n=3. SeeSupplementary Fig. 6for representative raw chromatograms. Figure 5: Ultraviolet laser DDFA of the pagC promoter region. Plasmid DNA containing the pagC region was incubated in the presence of 600 nM H-NS, 100 nM SlyA and 500 nM PhoP-P as indicated and exposed to a single pulse of 266 nm radiation. Crosslinking was quantified by fluorescent primer extension. The relative distance to the TSS is indicated in base pairs on the horizontal axis. Results are presented as DDFA plots, representing the difference in fluorescent peak height (relative fluorescent unit, RFU) between the protein-free control and the experimental sample ( a ). DDFA plots are also shown for the H-NS+SlyA, H-NS+PhoP-P and H-NS+SlyA+PhoP-P reactions representing the difference between the H-NS control and the experimental sample ( b ). Peaks represent a protein-induced change in DNA structure, typically owing to increased intramolecular contacts or DNA–protein crosslinks. Valleys also represent a change in DNA structure owing to decreased intramolecular contacts. Approximate sizes of peaks of note are indicated. Data represent the mean±s.d. ; n =3. See Supplementary Fig. 6 for representative raw chromatograms. Full size image The present study demonstrates that horizontally acquired genes are more likely to be regulated by counter-silencing than by the de novo evolution of a classical (group A) activation circuit, and that these mechanisms can be distinguished both architecturally and functionally. Classical PhoP-activated genes possess a precisely positioned PhoP-binding site overlapping the −35 box that allows PhoP to interact directly with RNAP ( Fig. 6 ), resembling a canonical class II-activated promoter [36] . In contrast, genes that are transcriptionally silenced by H-NS exhibit multiple architectures, indicating that counter-silencing has fewer structural constraints, as counter-silencing proteins need only antagonize endogenous silencing to achieve gene expression. These observations provide a mechanistic explanation for the variety of promoter architectures observed in bacteria. 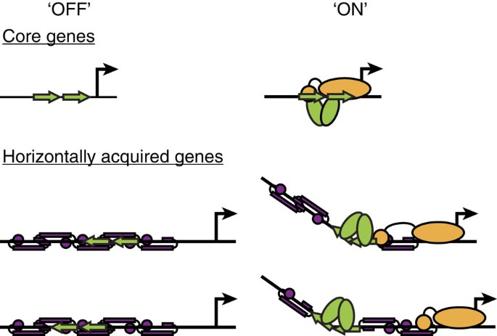Figure 6: Activation and counter-silencing are distinct mechanisms of transcription regulation. Activation occurs predominantly at core ancestral promoters, as it requires a precisely positioned and oriented activator binding site (green arrow) relative to the TSS (bent arrow). In its ‘ON,’ transcribed state, the promoter is bound by the activator, allowing a direct interaction with the RNAP (yellow) and an increase in transcription. Counter-silencing occurs at horizontally acquired genes, where the counter-silencer protein (green ovals) binds in a variety of positions and orientations. A silencing protein (purple) represses transcription in the ‘OFF’ state. In the transcribed ‘ON’ state, the counter-silencer binds local DNA, disrupting the structure of the silencing complex and recruiting the RNAP holoenzyme, allowing transcription. Figure 6: Activation and counter-silencing are distinct mechanisms of transcription regulation. Activation occurs predominantly at core ancestral promoters, as it requires a precisely positioned and oriented activator binding site (green arrow) relative to the TSS (bent arrow). In its ‘ON,’ transcribed state, the promoter is bound by the activator, allowing a direct interaction with the RNAP (yellow) and an increase in transcription. Counter-silencing occurs at horizontally acquired genes, where the counter-silencer protein (green ovals) binds in a variety of positions and orientations. A silencing protein (purple) represses transcription in the ‘OFF’ state. In the transcribed ‘ON’ state, the counter-silencer binds local DNA, disrupting the structure of the silencing complex and recruiting the RNAP holoenzyme, allowing transcription. Full size image Although classical activation was only observed for group A promoters under the experimental conditions used in this study, we concede that activation might also occur for group B promoters under certain conditions, as previous studies have suggested that group B promoters are subject to class I activation [19] . Furthermore the group B genes appear to be part of the core genome, as indicated by their average 47.5% AT content and their conservation in E. coli ( Table 1 ). However, we have no direct experimental evidence of activation at these promoters. The epistatic nature of the hns mutation in vivo ( Supplementary Fig. 2 ) suggests that an H-NS-dependent co-factor might be necessary for full activation at these promoters. Likewise, the significance of having multiple PhoP sites, as seen at the hybrid A/C and B/C promoters, is unclear. A single-group A site is capable of activating transcription, even in the presence of H-NS, as evidenced by orgB ( Supplementary Fig. 2 ), and the upstream site at the hybrid A/C virK promoter is dispensable for activation in transcript fusion experiments [19] , so the upstream site does not appear to be necessary for overcoming H-NS. Additional sites might also serve to increase the magnitude of the activator-dependent response or allow SlyA-independent counter-silencing by providing cooperativity between PhoP-P-bound sites. However, many of the hybrid promoters are regulated by SlyA, so this seems unlikely. A final possible explanation is that hybrid promoters represent evolutionary intermediates in the process of integrating genes into pre-existing regulatory circuitry. Upon initial integration into the host genome, they may have acquired a group C binding site and over time acquired additional sites through recombination. Ultraviolet laser footprinting suggests that H-NS alters the structure of the URR during silencing, most likely via stiffening [14] . Under counter-silencing conditions, SlyA and PhoP act cooperatively to remodel the H-NS–DNA complex at the URR, introducing a bend at the PhoP-binding site and restoring open-complex formation. As the URR is relatively distant from the promoter, two models for counter-silencing seem possible. The first is disruptive, wherein counter-silencers locally disrupt H-NS–DNA filament stiffening, perhaps via changes in DNA structure. This model is suggested by the DNA bend observed in the URR under counter-silencing conditions. The model is further supported by studies showing that filament formation is essential for silencing [35] , and that many proteins, such as the Lac and λ-repressors, are capable of counter-silencing in synthetic circuits [37] , presumably by disrupting H-NS polymerization and filament formation. The second possible pathway is supportive, wherein counter-silencers provide additional contacts for RNAP (possibly via its α-carboxyl terminal domain) to replace those otherwise occluded by H-NS. These supportive interactions could come in the form of either DNA–protein interactions, in which more distal DNA is brought closer to the RNAP by DNA bending, or protein–protein interactions, in which a counter-silencer such as PhoP-P directly interacts with RNAP, similar to class I activation [38] . This pathway is suggested by the observation that PhoP-P increases open-complex formation in the absence of H-NS ( Supplementary Fig. 7 ). Like class I activation, this model is likely to be dependent on the distance between the counter-silencer-binding sites and the TSS, as increasing the distance will decrease the probability that productive interactions will occur [39] . In either scenario, counter-silencing does not need to fully displace H-NS from the promoter but rather alters promoter structure to allow open-complex formation and productive transcription despite the presence of H-NS. It should also be noted that these models are not mutually exclusive, and it is likely that both occur in the cell. The observation that PhoP-P promotes open-complex formation at both pagC and phoP without the expected concomitant increase in transcription at pagC suggests that open-complex formation is not a rate-limiting step for the transcription of PhoP-P targets such as pagC in the absence of H-NS and implies that the rate-limiting step for group A activation is downstream of open-complex formation, likely at the stage of promoter escape when the holoenzyme undergoes many rounds of abortive transcript initiation before producing a full-length transcript. This may be a common phenomenon, as genome-wide analyses suggest that many silent promoters are bound by RNAP and ‘transcriptionally poised’ but not actively transcribed [33] . Structural analysis of PhoB, another OmpR-family response regulator, demonstrates that it can recruit RNAP to the promoter but must bind a site overlapping the −35 box in order to interact directly with the σ 70 domain 4 of the RNAP holoenzyme for full activation to occur [40] . This interaction remodels the holoenzyme and causes displacement of the linker between σ 70 domains 3 and 4, which otherwise blocks the RNA exit channel and promotes abortive transcript initiation by blocking promoter escape [41] . This could explain the precise positioning required for the PhoP box at group A promoters. PhoP must be correctly positioned in order to remodel the holoenzyme and allow promoter escape. In contrast, at silenced promoters, open-complex formation is completely inhibited and thus becomes the rate-limiting step in transcription, rather than promoter escape. It is notable that this pattern of PhoP-dependent regulation is lost when short linear DNA fragments are used as transcription templates ( Supplementary Fig. 5 ). Although small linear fragments are commonly used in molecular analyses of DNA–protein interactions, they do not appear to reliably recapitulate in vivo regulatory events in the case of PhoP. Thus, IVT analysis using linear DNA templates must be interpreted with caution. Counter-silencing by multiple factors, such as SlyA and PhoP, is not unique to pagC , as many PhoP targets are co-regulated by SlyA [42] , nor is it unique to the PhoP regulon, as other counter-silencing circuits such as csgD in E. coli have shown to be cooperatively regulated by multiple factors [43] . How cooperative regulation occurs is unknown, but there are at least two possible scenarios. In the first, multiple regulators such as SlyA and PhoP-P cooperatively remodel the bacterial chromatin by collaboratively increasing the affinity of each protein for its respective binding site to allow formation of a stable nucleoprotein complex. This requires binding sites for both proteins, most likely at a fixed position and orientation relative to each other. The promiscuous binding specificity of SlyA [44] makes it particularly suitable for such interactions. Collaborative binding has been reported at csgD , where integration host factor (IHF) binds cooperatively with OmpR and RstA to counter H-NS silencing [43] . Alternatively, two or more proteins may directly interact independently of DNA binding to form a complex with unique specificity and regulatory activity. However, in the case of pagC , SlyA and PhoP-P are each capable of binding the unprotected pagC promoter region independently of each other, and attempts to demonstrate a direct interaction between the two proteins have been unsuccessful [42] . Regardless of the mechanism, complex counter-silencing is functionally important as it provides a mechanism for signal integration [45] . Although several other cases of regulatory proteins acting via counter-silencing of H-NS have been reported, a detailed understanding of how these events relate to target promoter architecture has been lacking, making a structural distinction between counter-silencing and activation difficult. For example, the nucleoid-associated protein IHF counters H-NS silencing at the aforementioned csgD promoter in E. coli [43] , as well as the virF and icsA promoters in Shigella flexneri [46] . IHF is not thought to act as a classical transcriptional activator by interacting with RNAP but rather serves as an accessory architectural protein, bending DNA to facilitate contacts between RNAP and more distant upstream enhancers [47] . The pagC counter-silencer SlyA represses its own expression [48] as well as that of other conserved members of its regulon, but upregulates horizontally acquired [42] and H-NS-repressed [2] , [3] genes in S. Typhimurium. This suggests that SlyA was originally a transcriptional repressor that has evolved a role as a counter-silencer acting in concert with PhoP. Likewise, recent studies suggest that the LysR-type transcriptional regulator LeuO has evolved into a counter-silencer. SELEX (systematic evolution of ligands by exponential enrichment) experiments in E. coli suggest that 95% of LeuO targets are also bound by H-NS [49] , [50] . Although the fraction of co-regulated genes in S . Typhimurium (38%) appears to be much lower [51] , these findings suggest a significant role for LeuO in opposing H-NS. As with SlyA, the ability of LeuO to recognize DNA on the basis of shape rather than specific sequences make it an ideal counter-silencer. Proteins functionally analogous to H-NS have been described in diverse bacterial species including MvaT of P. aeruginosa [6] and Lsr2 of M. tuberculosis [5] , [52] , suggesting that silencing and counter-silencing are widespread regulatory mechanisms. However, it should also be noted that counter-silencing as a general mechanism is not only limited to H-NS targets but may also apply to other DNA-binding proteins capable of repressing transcription. Regulatory circuits fitting this model have been described for regulatory factors such as NarL/NarP-mediated counter-silencing of IHF at the nrf promoter in E . coli [53] . Our analysis of the S. Typhimurium PhoP regulon suggests that counter-silencing may be among the most common mechanisms of transcription regulation in bacteria. This is likely to result from its architectural flexibility that facilitates the expansion of regulatory networks by horizontal gene transfer and underscores the fundamental importance of counter-silencing in bacterial evolution. General protocols Plasmid DNA for all biochemical assays was purified using a Midi kit (Qiagen, Valencia, CA), following the manufacturer’s protocol for very low copy plasmids. The resulting product was further purified by extraction with phenol:CHCl 3 :IAA (25:24:1) twice, followed by ethanol precipitation and two washes with 70% ethanol. DNA pellets were dissolved in 10 mM Tris-HCl (pH 8.0), and stored in aliquots at −20 °C. DNA for all other protocols was purified using a Mini kit (Qiagen). All oligonucleotides used in this study are described in Supplementary Table 1 . Strain construction All Salmonella enterica serovar Typhimurium strains were constructed in a 14028s rpoS low genetic background, which is required for the viability of hns mutant strains [2] . The slyA::Cm deletion mutant was generated with primers WNp291 and WNp292 using the λ-Red recombinase protocol [54] . The hns mutant strain, WN342, has been previously described [2] . The phoP mutant strain was generated by transferring the phoP105 ::Tn 10 d cassette from TT13208 (ref. 55 ) into 14028s rpoS low via P22HT int -mediated transduction. The hns slyA , hns phoP and slyA phoP double mutants, and the hns slyA phoP triple mutant were constructed by introducing the cassettes described above into 14028s rpoS low via P22HT int -mediated transduction. qRT–PCR analysis of in vivo gene expression Overnight cultures in Luria Bertani (LB) broth were diluted 1:100 in LB broth and grown to OD 600 ~0.6, pelleted and washed twice in N -minimal medium containing 10 mM MgSO 4 or 10 μM MgSO 4 , then resuspended in the indicated N -minimal medium and incubated for 30 min at 37 °C with shaking. Cells were then pelleted and resuspended in TRIzol reagent (Life Technologies, Grand Island, NY) and incubated for a minimum of 30 min. RNA was then purified following manufacturer’s instructions. Residual DNA was removed by digestion with 5 U DNase I (Thermo Fisher Scientific, Pittsburgh, PA), followed by extraction with acid-phenol:chloroform (1:1). RNA was precipitated in 95% ethanol and the resulting pellet was dissolved in RNase-free water. RNA was converted to cDNA using RevertAid reverse transcriptase (Thermo Fisher Scientific) and RiboLock RNase inhibitor using random hexamers (IDT, Coralville, IA) according to the manufacturer’s recommendations. qPCR was performed in a Rotor-Gene 3000 (Qiagen) using SYBR green master mix [56] . The pagC , phoP and rpoD transcripts were quantified using oligonucleotide pairs SLP1000/SLP1001, phoP-F/phoP-R, and SLP1010/SLP1011, respectively. The mgtA , orgB , pmrD , ompX , rstA , mgtC , pagK , pgtE and ugtL transcripts were quantified with oligonucleotide pairs mgtA-F/mgtA-R, orgB-F/orgB-R, pmrD-F/pmrD-R, ompX-F/ompX-R, rstA-F/rstA-R, mgtC-F/mgtC-R, pagK-F/pagK-R, pgtE-F/pgtE-R and ugtL-F/ugtL-R, respectively. The relative expression of all PhoP regulon members was determined for each sample by first normalizing expression levels relative to rpoD transcript, then normalizing relative to the wild-type non-induced (10 mM MgSO 4 ) sample for that experimental replicate. Cloning Plasmid pRW6 was constructed by cloning a 2.7-kb PCR fragment generated from primers pagC(2.7)-F and pagC(2.7)-R into the BamHI and EcoRV sites of pWKS30 (ref. 57 ). Plasmid pRW9 was constructed by cloning a 2.4-kb PCR fragment containing the pmrD gene generated from primers pmrD(2.4)-F and pmrD(2.4)-R into the BamHI and EcoRV sites of pWKS30. Plasmid pRW11 was constructed by cloning a 2.7-kb PCR fragment generated from primers phoP(2.7)-F and phoP(2.7)-R into the EcoRI and BamHI sites of pWKS30. Plasmid pRW12 was constructed by cloning a (1.8-kb) PCR fragment containing the entire ugtL gene generated from primers ugtL(1.8)-F and ugtL(1.8)-R into the EcoRI and BamHI sites of pWKS30. Plasmid pRW13 was constructed by cloning a PCR fragment generated from primers his-hns-F and hns-R into the NcoI and XbaI sites of pTRC99a (ref. 58 ). Plasmid pRW14 was constructed by cloning a PCR fragment generated from the primers phoP-his-F and phoP-his-R into the KpnI and XbaI sites of pBAD18 (ref. 59 ). Plasmid pRW14 was generated by cloning a 1.7-kb PCR fragment of the rstA region, amplified using primers EcoRI-rstA-F and BamHI-rstA-R into the EcoRI and BamHI sites of pWKS30 (ref. 57 ). Plasmid pRW20 was generated by cloning tR2 (ref. 60 ) and t500 (ref. 61 ) transcription terminators into the multiple cloning site of pWKS30, and deleting its lac promoter. The t500 terminator was cloned into the KpnI and XhoI sites using double-stranded DNA (5′- GCCGCCGGTACCCAAAGCCCGCCGAAAGGCGGGCTTTTCTGTCTCGAGGCCGCC -3′) synthesized by IDT. The tR2 terminator was cloned into the SacI and XbaI sites using double-stranded DNA (5′- GCCGCCGAGCTCAACAGGCCTGCTGGTAATCGCAGGCCTTTTTTTTCTAGAGCCGCC -3′) synthesized by IDT. The lac promoter was deleted using the QuikChange mutagenesis protocol (Agilent Technologies, Santa Clara, CA) and oligonucleotides lac-prom-del-F and lac-prom-del-R. Plasmids pRW23 and pRW28 were generated using the QuikChange mutagenesis protocol (Agilent Technologies). Plasmid pRW23 contains a mutant pagC -10 box (5′- CGCGGC -3′), generated using the primers pagC-10-mut-F and pagC-10-mut-R. Plasmid pRW28 features a 20-bp deletion of the phoP TSS and −10 box; the −35 box and PhoP-binding site were retained. Plasmid pRW30 was generated by cloning a 4.7-kb fragment of the mgtA region, amplified using the primers BamHI-mgtA-F and HindIII-mgtA-R into the BamHI and HindIII sites of pWKS30 (ref. 57 ). Plasmid pRW31 was generated by cloning a 2.1-kb fragment of the orgB region, amplified using the primers BamHI-orgB-F and HindIII-orgB-R into the BamHI and HindIII sites of pWKS30 (ref. 57 ). Plasmid pRW32 was generated by cloning a 2.5-kb fragment of the pagK region, amplified using the primers BamHI-pagK-F and EcoRI-pagK-R into the BamHI and EcoRI sites of pWKS30 (ref. 57 ). Plasmid pRW33 was generated by cloning a 3.2-kb fragment of the pgtE region, amplified using the primers BamHI-pgtE-F and HindIII-pgtE-R into the BamHI and HindIII sites of pWKS30 (ref. 57 ). Plasmid pRW34 was generated by cloning a 3.7-kb fragment of the mgtC region, amplified using the primers BamHI-mgtC-F and EcoRI-mgtC-R into the BamHI and EcoRI sites of pWKS30 (ref. 57 ). Plasmid pRW35 was generated by cloning a 4.0-kb fragment of the ompX region, amplified using the primers HindIII-ompX-F and BamHI-ompX-R into the HindIII and BamHI sites of pRW20. Purification of H-NS H-NS was purified as an N -terminal 6 × His-tagged protein expressed from pRW13. E. coli BL21(DE3) pLysS/pRW13 was grown in 2 l LB broth to 0.7 OD 600 at 37 °C then induced with 1 mM isopropyl β- D -thiogalactoside for 3 h. Cells were harvested via centrifugation and stored at −80 °C for subsequent processing. Cell pellets were suspended in 30 ml lysis buffer (50 mM NaH 2 PO 4 , 300 mM NaCl and 10 mM imidazole, pH 8.0), containing 1 mg ml −1 lysozyme and complete EDTA-free protease inhibitors (Roche Applied Science, Penzberg, Germany). Suspensions were mixed on ice for 45 min and then lysed by sonication. Lysates were centrifuged three times for 30 min at 10,000 r.p.m. and 4 °C. The cleared lysate was applied to a 5-ml HisTrap HP column (GE Healthcare, Piscataway, NJ), washed extensively with wash buffer (50 mM NaH 2 PO 4 , 300 mM NaCl and 20 mM imidazole, pH 8.0), then eluted over a linear gradient of elution buffer (50 mM NaH 2 PO 4 , 300 mM NaCl and 500 mM imidazole, pH 8.0). Fractions containing H-NS were pooled and dialysed into PE buffer (10 mM potassium phosphate (pH 7.5), 1 mM EDTA and 10 mM β-mercaptoethanol). This material was applied to a HiTrap Heparin column (GE Healthcare) and eluted using a 125-ml linear gradient of PE containing 1 M NaCl. Samples were pooled and concentrated using an Amicon Ultracel-4 centrifugal concentrator (EMD Millipore, Billerica, MA), then dialysed into 10 mM potassium phosphate (pH 7.5), 200 mM NaCl, 50% glycerol, 1 mM dithiothreitol (DTT). Approximate protein concentrations were determined via absorbance at 280 nm, and individual protein preparations were normalized relative to specific activity (silencing activity). Purified protein was stored in aliquots at −80 °C. Activity of the construct in vivo was confirmed by complementation of an hns mutant strain. Purification of PhoP PhoP was purified as a C-terminal 6 × His-tagged protein expressed from pRW14. E. coli BL21(DE3)/pRW14 was grown in LB broth to 0.7 OD 600 and induced by the addition of 0.2% arabinose. Cells were then grown and harvested as described for H-NS. Protein was purified on a HisTrap HP column (GE Healthcare) as described for H-NS, but following elution, fractions containing PhoP were identified via A 280 and SDS–polyacrylamide gel electrophoresis, pooled, dialysed into PhoP storage buffer (50 mM Tris-HCl (pH 7.5), 200 mM KCl, 10 mM MgCl 2 , 0.1 mM EDTA, 1 mM DTT and 50% glycerol), and concentrated using an Amicon Ultracel-10K centrifugal concentrator (EMD Millipore). Approximate protein concentrations were determined via absorbance at 280 nm, and individual protein preparations were normalized relative to specific activity (activation and counter-silencing activities). Purified protein was stored in aliquots at −80 ° C. Purification of SlyA SlyA was purified as an N -terminal 6 × His-tagged protein from pET16B:: slyA [42] , essentially as described for H-NS above, except that following elution from the HiTrap Heparin (GE Healthcare) column, the material was dialysed in 20 mM Tris (pH 7.6), 150 mM NaCl, 0.1 mM EDTA, 5 mM DTT and 50% glycerol, and stored in aliquots at −80 ° C. Approximate protein concentrations were determined via absorbance at 280 nm, and individual protein preparations were normalized relative to specific activity (that is, counter-silencing activity). Phosphorylation of PhoP PhoP was phosphorylated by incubating 20 μM PhoP in phosphorylation buffer (50 mM Tris-HCl (pH 7.6), 200 mM KCl, 0.1 mM EDTA, 5 mM MgCl 2 and 5% glycerol) with 25 mM acetyl phosphate for 3 h at room temperature. Unphosphorylated PhoP was incubated for 3 h in phosphorylation buffer without acetyl phosphate. Protein was then stored on ice and used within 2 h. In vitro transcription Reactions were assembled in IVT buffer containing 40 mM HEPES, pH 7.3, 60 mM potassium glutamate, 1.5 mM MgCl 2 , 0.5 mM CaCl 2 , 1 mM DTT, 0.05% NP-40, 0.1 mg ml −1 BSA and 10% glycerol to a final volume of 20 μl. The appropriate template was added, as indicated in Supplementary Table 2 , to a final concentration of 1 nM, followed by 20 U of recombinant RNasin (Promega, Madison, WI). Reactions were allowed to equilibrate at room temperature, appropriately diluted H-NS, SlyA or PhoP were added as indicated, and the reaction incubated for an additional 10 min. For counter-silencing reactions, H-NS was first added and the reaction was incubated for 10 min before addition of SlyA or PhoP, after which the reaction was incubated for another 10 min. RNAP holoenzyme (Epicentre, Madison, WI) was then added to a final concentration of 10 nM and the reaction was incubated for 10 min before rNTPs were added to a final concentration of 1 mM. The transcription reaction was incubated for 20 min at room temperature before stopping by the addition of 20 μl of DNase I buffer containing 10 mM Tris-HCl (pH 7.5), 2.5 mM MgCl 2 , 0.1 mM CaCl 2 and 4 U of DNase I (Thermo Fisher Scientific) and incubation for 30 min at 37 °C. EDTA was added to a final concentration of 5 mM and DNase I was inactivated by incubating the reaction at 65 °C for 5 min. Reactions were then chilled on ice and were diluted appropriately with H 2 O to bring them within the linear range of the detection protocol. IVT reactions were quantified via RT–PCR using strand- and sequence-specific probes to ensure unambiguous quantification of the transcript of interest. cDNA was generated using the QuantiTect RT–PCR kit (Qiagen) following the manufacturer’s instructions, with the following modifications: sequence-specific oligonucleotide probes were used as indicated in Supplementary Table 2 , instead of the manufacturer’s primer mix, and the synthesis step was allowed to proceed for 30 min. Reactions were quantified via qPCR, as described above, using the same primer pairs as described for qRT–PCR, except for mgtA , where the primer pair mgtA-IVT-F/mgtA-IVT-R was used, and pagC , where pagC-3′-F/pagC-3′-R was used. Absolute reaction output was determined using a standard curve of each PCR product. KMnO 4 footprinting Reactions were assembled as described for IVT reactions, except that DTT was omitted from the IVT buffer, and RNasin and rNTPs were not added. Ten nanomolar RNAP, 600 nM H-NS, 100 nM SlyA and 500 nM PhoP-P were added as indicated. Following assembly of the DNA–protein complexes, KMnO 4 was added to a final concentration of 2 mM, and the reaction was allowed to proceed for 2 min. Reactions were stopped by the addition of 2 μl of 14 M β-mercaptoethanol, followed by 78 μl quench buffer containing 1 M β-mercaptoethanol, 20 mM EDTA and 385 mM sodium acetate (pH 7.0). Reactions were then extracted with phenol:CHCl 3 :IAA (25:24:1), ethanol precipitated after the addition of 2 μl glycogen, washed twice in 70% ethanol, dried and re-dissolved in 20 μl H 2 O. Reactions were detected via fluorescent primer extension (described below). Ultraviolet laser footprinting Reactions were performed based on a protocol described elsewhere [34] , [62] . In brief, ultraviolet irradiation of DNA produces photoreactions, predominantly pyrimidine dimers (although protein–DNA crosslinks can also form), as a function of DNA conformation and protein binding. Reactions were assembled as described for IVT reactions, except that RNasin, RNAP and rNTPs were omitted. Reactions were assembled in 0.2 ml tubes with optically clear (Bio-Rad, Hercules, CA) caps to allow transmission of the laser beam. Tubes were placed in a custom-machined black polycarbonate pedestal to absorb scattered laser light and exposed to an average of one 10 ns pulse of ultraviolet radiation at 266 nm, with an output pulse energy of ~10 mJ. Pulses were generated using the fourth harmonic of a Q-switched Nd:YAG laser (Spectra-Physics Quanta-Ray GCR-170; Spectra-Physics, Santa Clara, CA). Exposures were controlled using an SH05 Optical Beam shutter and a SC10 Shutter controller (Thorlabs, Newton, NJ). Following exposure, samples were immediately placed on crushed dry ice and stored at −80 °C until processed. Samples were brought to a volume of 100 μl in 300 mM sodium acetate (pH 7.0) and 0.2 mg ml −1 proteinase K, and incubated at 50 °C for 5 min. Reactions were then extracted and precipitated as described for KMnO 4 footprinting, and analysed using fluorescent primer extension (described below). DNase I footprinting Reactions were assembled as described for ultraviolet laser footprinting. Following protein binding, 0.005 U DNase I (Thermo Fisher Scientific) were added and each reaction was digested for 2 min. Under these conditions, each plasmid is nicked approximately once per molecule. The footprinting reaction product is therefore, on average, representative of binding to supercoiled DNA. Each digestion was stopped by the addition of 180 μl cold stop buffer containing 330 mM sodium acetate (pH 7.0), 20 mM EDTA and 0.5% sarkosyl, vortexed and placed on ice. Samples were extracted and precipitated as described for KMnO 4 footprinting and detected using fluorescent primer extension (described below). Fluorescent primer extension Fluorescent primer extension was performed in 50 μl reaction volumes using the entire footprinting reaction product. Each reaction contained 1 × ThermoPol Buffer (New England Biolabs), 0.1 mM dNTPs, 40 nM 5′ 6-FAM-labelled primer and 1 U Vent R (exo − ) DNA polymerase (New England Biolabs). The pagC samples were analysed using the primer 6FAM-pagC. Reactions were denatured for 3 min at 95 °C followed by 70 cycles of 1 min at 95 °C, 1 min annealing at 51 °C and 1 min extension at 72 °C. Reactions were purified using SigmaSpin sequencing clean-up columns (Sigma-Aldrich, St Louis, MO) according to the manufacturer’s instructions, dried and dissolved in 20 μl H 2 O. Reactions were analysed on an Applied Biosystems 3730xl DNA Analyzer at the Fred Hutchinson Cancer Research Center Genetic Analysis Lab (Seattle, WA). Differential DNA footprint analysis DDFA is a differential sensitivity method for analysing footprinting data adapted from a technique described by Joshi et al . [63] Samples were run on an ABI 3730xl DNA Analyzer with GeneScan 500 LIZ size standards (Life Technologies). Analysis was performed using a modified AFLP analysis method in GeneMapper 4.0 (Life Technologies). First, a custom set of size standard definitions was generated, omitting the 35-bp and 250-bp standards, to allow the software to correctly size-call the samples. For the DNase I and ultraviolet laser footprinting reactions, all replicates were analysed as a group to ensure similar sizing and normalization, and normalized to the sum of total fluorescence over the entire project with light smoothing. KMnO 4 samples were not normalized owing to high degree of variability in fluorescence inherent to the protocol. A panel was then generated using all samples with a bin width of 0.5 bp. Size-calling was performed using the local Southern method. Minimum peak half width was set to 2 points, a polynomial degree of 5 and a peak window size of 7 points. Maximum peak width was set to 1 bp. Peak height data was then exported to Excel (Microsoft, Redmond, WA) for analysis. Peak height, rather than peak area, was used owing to the high resolution (1 bp) of this data, as it was judged to be more accurate. Missing peak data, which is inherent in samples or regions with a low baseline signal or poorly defined peaks, was determined manually in the GeneMapper software. Bases with no detectable peak were assigned a peak height of 35 relative fluorescent units, which is approximately equal to the baseline. Replicates with poor size-calling were discarded. Sizing was manually adjusted to correct for variability in fragment mobility. Differential sensitivity was then determined by subtracting peak height data for the relevant control from the experimental sample. In the case of DNase I footprinting, this results in a valley for protected or bound sites, and peaks in the case of exposed sites, typical of bent DNA. In the case of ultraviolet laser footprinting, valleys suggest decreased intramolecular contact between bases, whereas peaks indicate increased contact or DNA–protein crosslinks. Peaks in KMnO 4 samples indicate regions of single-stranded DNA. Difference analysis replicates were exported to GraphPad Prism (GraphPad Software, San Diego, CA), where the means and s.d.’s were determined and plotted relative to the TSS. All plots represent the mean of at least three replicates. How to cite this article: Will, W. R. et al . Evolutionary expansion of a regulatory network by counter-silencing. Nat. Commun. 5:5270 doi: 10.1038/ncomms6270 (2014).